Molecular origins of internal friction effects on protein-folding rates Recent experiments on protein-folding dynamics have revealed strong evidence for internal friction effects. That is, observed relaxation times are not simply proportional to the solvent viscosity as might be expected if the solvent were the only source of friction. However, a molecular interpretation of this remarkable phenomenon is currently lacking. Here, we use all-atom simulations of peptide and protein folding in explicit solvent, to probe the origin of the unusual viscosity dependence. We find that an important contribution to this effect, explaining the viscosity dependence of helix formation and the folding of a helix-containing protein, is the insensitivity of torsion angle isomerization to solvent friction. The influence of this landscape roughness can, in turn, be quantitatively explained by a rate theory including memory friction. This insensitivity of local barrier crossing to solvent friction is expected to contribute to the viscosity dependence of folding rates in larger proteins. Interpreting experiments and simulations on protein folding appears at the outset to be a daunting task given the large number of degrees of freedom involved. Nonetheless, both in experiment and simulation, it is common to model the dynamics of this complex process as diffusion along a single reaction coordinate, an approach motivated by the energy landscape theory for protein folding [1] , [2] , [3] , [4] . From this perspective, diffusion along the folding coordinate is controlled both by the solvent viscosity and by the roughness of the landscape, that is, local barriers such as those arising from dihedral angle rotations or the making/breaking of interatomic contacts [5] , [6] . Experimentally, it is possible to probe these contributions by varying solvent viscosity. If the diffusion coefficient for protein dynamics is determined mainly by movement of the chain through the solvent, then overall folding rates might be expected to be inversely related to the solvent viscosity, if the chain diffusion follows Stokes’ law. Deviations of protein-folding rates from Stokes-like behaviour would then suggest that not only solvent friction is important but that a contribution from the protein, known as ‘internal friction’, plays a role [7] , [8] , [9] , [10] , [11] . Following pioneering work quantifying viscosity-dependent dynamics and internal friction in folded proteins [7] , [12] , evidence for internal friction has recently been found in protein folding [10] , [13] , [14] , [15] , [16] , [17] , [18] , the chain dynamics of unfolded states or disordered proteins [19] and even in small peptides [13] , [20] , [21] , making it a ubiquitous theme in the study of protein dynamics. The problem has also been tackled using simulation and theory [5] , [6] , [19] , [21] , [22] , [23] , [24] , [25] . Even so, a molecular-level description for the deviation of the rates from the inverse scaling with viscosity is still lacking [26] , with internal friction generally being described at a phenomenological level. The only study to model the solvent in molecular detail concluded that breaking and formation of hydrogen bonds appeared to be the most likely cause of internal friction in peptides [21] . Here, we use molecular dynamics simulations in explicit solvent to demonstrate an important contribution towards deviations from k ∝ 1/ η , helping to explain many experimental observations. We find that simulations of a number of different peptides and proteins exhibit a similar deviation from first-power dependence of relaxation time on solvent viscosity. These include all-atom models of a minimal helix-forming peptide, a peptide used in contact formation experiments and a 20-residue mini-protein, and coarse-grained simulations of a fast-folding helical protein. In cases where comparable experimental data are available, we obtain excellent agreement. In order to probe the origin of this effect, we have considered simpler systems, which enable us to probe possible contributions to the dependence of folding rates on solvent viscosity. Our main finding is that local roughness of the energy landscape can give rise to apparent internal friction effects due to the insensitivity of local barrier crossing events to solvent viscosity. This explains the deviations from inverse viscosity dependence of relaxation rates observed in the dynamics of helix formation, and for the folding of some helical proteins. However, it is likely that the much stronger internal friction observed for the folding of some proteins [10] and for unfolded protein dynamics at low denaturant concentrations [19] may have additional causes. Internal friction in peptide and protein dynamics As our first example for investigating viscosity-dependent folding rates, we use a short helix-forming peptide, as α-helices are the smallest peptides for which deviations from inverse first-power viscosity dependence have been observed experimentally [13] , and we can thoroughly sample the dynamics of this system in molecular simulations. We study the five-residue blocked Ala 5 , using unbiased all-atom simulations in explicit water ( Fig. 1a ) at constant temperature and pressure. In experiments, viscosity is usually varied by adding viscogenic agents such as glycerol or sucrose to the solution. This may have the undesirable effect of modifying the free energy surface of the protein, which must be approximately compensated by adding chemical denaturants [27] . In simulations, we can carry out an idealized change of viscosity, which has no effect on the free energy surface, thus simplifying the interpretation of the resulting dynamics. This is achieved by scaling the masses of the water molecules, effectively rescaling time: scaling the masses by a factor of α translates into an α 1/2 scaling of the viscosity of pure water [21] , [28] . This method has recently been used in a study of the Ala 8 and (GlySer) 4 peptides, which revealed internal friction effects, even for these simple systems [21] . In Supplementary Fig. 1 , we confirm that the shear viscosity of the pure solvent computed using the Green–Kubo relation shows the expected dependence on solvent mass. We have thus scanned a wide range of viscosities by running a series of simulations of Ala 5 using different masses for the water molecules. 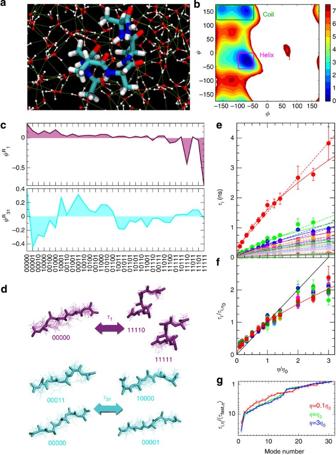Figure 1: Peptide dynamics in explicit water. (a) Ala5(thick lines) in water, hydrogen bonds indicated by broken lines. (b) Ramachandran free energy surface averaged over all backboneϕ,ψtorsion angles in Ala5. Units of energy arekBT. Squares mark the core regions used for the assignment of simulation trajectories to coarse states. (c) Right eigenvectors for the slowest and fastest eigenmodes, corresponding to helix formationand equilibration within the coil state. (d) Examples of states with large weight in the eigenvectors from (c). (e) Viscosity dependence of all 31 relaxation times in Ala5. Solid lines are fits to a power-law and broken lines are linear fits. (f) Viscosity-dependent relaxation times normalized to the relaxation time at normal water viscosity. Solid red line is the power-law fit to the slowest relaxation and solid black line represents an ideal first-power dependence of relaxation time on viscosity. Errors bars were obtained from bootstrap tests. (g) Mode spectrum of Ala5for different solvent viscosities as indicated. All timescales have been divided by the average relaxation time of the 10 fastest modes at each viscosity. Full details of the simulation parameters for the different solvent masses and peptides are given in Supplementary Table 1 . We have confirmed that the equilibrium distribution, quantified by the distribution of RMSD from a helix, is the same for all solvent viscosities ( Supplementary Fig. 2 ). Figure 1: Peptide dynamics in explicit water. ( a ) Ala 5 (thick lines) in water, hydrogen bonds indicated by broken lines. ( b ) Ramachandran free energy surface averaged over all backbone ϕ , ψ torsion angles in Ala 5 . Units of energy are k B T . Squares mark the core regions used for the assignment of simulation trajectories to coarse states. ( c ) Right eigenvectors for the slowest and fastest eigenmodes, corresponding to helix formation and equilibration within the coil state . ( d ) Examples of states with large weight in the eigenvectors from ( c ). ( e ) Viscosity dependence of all 31 relaxation times in Ala 5 . Solid lines are fits to a power-law and broken lines are linear fits. ( f ) Viscosity-dependent relaxation times normalized to the relaxation time at normal water viscosity. Solid red line is the power-law fit to the slowest relaxation and solid black line represents an ideal first-power dependence of relaxation time on viscosity. Errors bars were obtained from bootstrap tests. ( g ) Mode spectrum of Ala 5 for different solvent viscosities as indicated. All timescales have been divided by the average relaxation time of the 10 fastest modes at each viscosity. Full size image The dynamics of helical peptides is often poorly described by a simple two-state kinetic model [29] , [30] , [31] . We have therefore used a Markov state model (MSM) to characterize the helix-coil dynamics. Briefly, this is a discrete Markovian model in which the peptide exchanges among a finite set of chosen states. In this case, by defining each residue as being either ‘helical’ or ‘coil’ using its backbone torsion angles ( Fig. 1b ), we obtain a total of 32 possible global states for the peptide. The kinetics of interconversion of these states is described using an MSM derived from the simulation trajectory data, as described in the Supplementary Methods . The choice of backbone torsion angles to define states is justified by the fact that these are the most obvious slow degrees of freedom present, and indeed such MSMs have previously been successfully applied to the dynamics of this peptide [32] , [33] . A further advantage of using the MSM approach here, as opposed to, for example, projection of dynamics onto a reaction coordinate, is that it allows us to resolve the influence of solvent viscosity on microscopic relaxation modes (fast timescales) as well as on the global peptide-folding dynamics (slow timescales). For example, the eigenvectors for the slowest and fastest modes are shown in Fig. 1c . These eigenvectors contain the weights for the exchange of each state at the corresponding time scale. Clearly, for the slowest mode ( τ 1 ) the associated process corresponds to the interconversion of helix and coil states, while the fastest mode ( τ 31 ) involves exchange among various coil states, as illustrated by the structures with largest weights in these modes shown in Fig. 1d . By repeating this analysis for independent simulations of the peptide in water models with rescaled masses, we obtain the viscosity dependence of all 31 non-stationary eigenvalues of the kinetic model ( Fig. 1e ). As viscosity is increased, there is a general increase in all of the relaxation times of the model. Although the kinetic analysis at each viscosity was performed independently, the errors are small enough to determine the viscosity dependence of the relaxation times. It is immediately evident that all the relaxation timescales deviate from a first-power dependence on solvent viscosity. Linear fits of viscosity dependence of the relaxation times ( τ i ,η ) yield non-zero intercepts of different magnitudes for different modes. For the slowest mode the extrapolated relaxation time at η =0, τ 1, η =0 , is 0.35 ns, consistent with the extrapolated folding timescales previously reported for Ala 8 and (GlySer) 4 (ref. 21 ). The data are also well fitted by an empirical power-law expression τ = τ 0 ( η / η 0 ) β , with exponents β ranging from 0.45 to 0.75; here, we take the reference viscosity η 0 to be that when the water molecules have their standard mass. For the fast and slow modes, β clusters around 0.57 and 0.65, respectively. These values of β are very close to that reported for experiments on an α-helix-forming peptide, 0.64 (ref. 13 ). Both the linear and power-law fits are treated here as phenomenological. In previous studies, the data could often be fitted equally well by both functions [13] , [21] . However, there are some examples where only a power-law fit is adequate [34] , and there is more theoretical support for this functional form, as discussed further below [35] , [36] . Therefore, we have primarily used power-law fits to characterize our results. To compare the viscosity dependence of the different eigenmodes, we normalize their relaxation times by the fitted time at the normal viscosity of the water model, η 0 ( Fig. 1f ). Remarkably, we find that the normalized timescales τ i ,η0 for all 31 non-stationary eigenmodes i of the MSM of Ala 5 exhibit a similar deviation from the ‘zero-internal friction’ behaviour (that is, the 1:1 line). This result indicates that, regardless of the type of transition described by the mode (that is, global folding in the case of the slowest modes and local dihedral rotations for the fast modes, in the current discretization), a similar effect is observed, suggesting a common origin. Note that there is a systematic difference between the fast and slow modes, with the faster modes being generally less sensitive to solvent viscosity ( Fig. 1g ), a point to which we return below. We explore the generality of this observation by performing analogous simulations for several other peptide and protein systems. As an example of a highly disordered peptide, we chose the sequence C(AGQ) 2 W-NH 2 , which has been used as to probe the dynamics of contact formation via the quenching of the triplet state of the tryptophan by the cysteine [37] . In Fig. 2a we show two descriptors of the dynamics in this peptide: the slowest time-scale for an MSM constructed in the same way as for the Ala 5 peptide, and the diffusion-limited rate of Cys-Trp contact formation. The latter quantity corresponds to the rate of tryptophan quenching if every collision with the cysteine resulted in quenching, and thus depends only on the peptide dynamics. Both dynamical descriptors scale similarly with solvent viscosity. Furthermore, the results for this system suggest that the observed viscosity scaling is not limited to alanine-based peptides [21] . 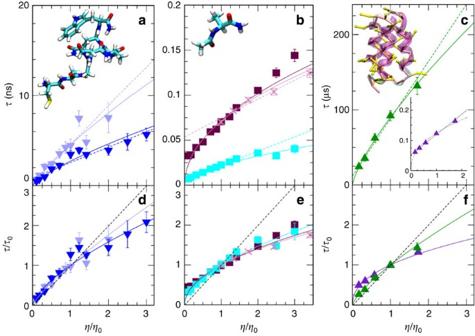Figure 2: Variation of relaxation times with water viscosity for different molecules. (a) C(AGQ)2W peptide: slowest relaxation mode (light triangles) from the MSM and diffusion-limited Trp-Cys contact formation time (dark triangles) (b) Alanine dipeptide: relaxation times for the standard force-field (violet squares) and for a version in which the barrier for rotation about theψtorsion angle has been lowered by ~5 kJ mol−1(cyan squares). Relaxation times from simulations in which viscosity was varied by adding glucose, rather than altering solvent mass, are shown in by purple crosses. (c) Coarse-grained protein model21: two-state folding relaxation time; inset: relaxation time for torsional transitions for an Ala4molecule in the same force field. Solid and dashed lines in upper panels are, respectively, power-law and linear fits. (d–f) Relaxation timesτinormalized by the value of the power-law fit at the normal water viscosity of the model corresponding toa–c, respectively. Normalized power-law fits are also shown. In all cases errors bars were obtained from bootstrap tests. Figure 2: Variation of relaxation times with water viscosity for different molecules. ( a ) C(AGQ) 2 W peptide: slowest relaxation mode (light triangles) from the MSM and diffusion-limited Trp-Cys contact formation time (dark triangles) ( b ) Alanine dipeptide: relaxation times for the standard force-field (violet squares) and for a version in which the barrier for rotation about the ψ torsion angle has been lowered by ~5 kJ mol −1 (cyan squares). Relaxation times from simulations in which viscosity was varied by adding glucose, rather than altering solvent mass, are shown in by purple crosses. ( c ) Coarse-grained protein model [21] : two-state folding relaxation time; inset: relaxation time for torsional transitions for an Ala 4 molecule in the same force field. Solid and dashed lines in upper panels are, respectively, power-law and linear fits. ( d – f ) Relaxation times τ i normalized by the value of the power-law fit at the normal water viscosity of the model corresponding to a – c , respectively. Normalized power-law fits are also shown. In all cases errors bars were obtained from bootstrap tests. Full size image Having obtained a similar viscosity dependence in all-atom simulations of two different peptides, we studied the prototypical polypeptide dihedral transition, namely the isomerization of alanine dipeptide. A two-state model of alanine dipeptide with the same discretization of the Ramachandran map as for Ala 5 , yields a very similar viscosity dependence of the relaxation time ( Fig. 2b ). After normalization by the relaxation time at normal water viscosity, the viscosity dependence of the alanine dipeptide relaxation closely resembles those for the other peptides, with a slightly smaller power-law exponent ( Fig. 2e ). This strongly suggests that the source of the apparent internal friction in the peptides considered is rotation about dihedral angles. We also consider, for this simplest example, the result of varying solvent viscosity by adding the viscogen glucose (used in experimental work on both helical peptides [13] and proteins [15] ), rather than by changing the solvent mass (details in Supplementary Methods and Supplementary Fig. 3 ). Remarkably, we find that over the range of glucose concentrations where the free energy surface of alanine dipeptide appears unaffected ( Supplementary Fig. 4 ), changing the solvent viscosity by addition of viscogens has an almost identical effect on the rates to the scaling of solvent mass ( Fig. 2b ). This suggests that isomerization of dihedral angles is a source of the deviation from first-power viscosity dependence of relaxation times both in experiments, where chemical viscogens are added, and in our simulations, where solvent mass is scaled. So far, we have considered relatively small peptides and so the internal friction effects may not be representative of the folding dynamics of larger proteins. Since sampling even a handful of protein-folding events with explicit solvent is still a challenging computational task, we adopt a previously described coarse-grained folding model [21] : briefly, it is a Gō-like folding model in an explicit coarse-grained solvent, with approximately two-state kinetics. As an example of a single torsion angle transition in this model, we also consider a Martini model for the peptide Ala 4 . We compute the folding time of the protein and the relaxation time for dihedral isomerization for the coarse-grained Ala 4 model as a function of solvent viscosity ( Fig. 2c ). Both timescales show clear evidence of internal friction effects. Normalization of these times using the times at normal water viscosity reveals that the internal friction effects are slightly weaker for the whole protein than for the Ala 4 model, a trend which is qualitatively similar to that for the all-atom models ( Fig. 2g ). The most likely origin of the more Stokes-like viscosity dependence for the protein is that folding dynamics is more strongly influenced by diffusion of the helices through the solvent. This mechanism is supported by the relatively high helix propensity of the protein in the unfolded state, such that both diffusion of helices and helix formation are relevant to folding. Microscopic origin of viscosity dependence We have shown clear evidence for a deviation from first-power viscosity dependence of relaxation times in a variety of systems. Since the scaling of the dynamics with solvent viscosity is fairly similar in all cases, a possible explanation could be a breakdown of Stokes Law due to the comparable sizes of solute and solvent. The breakdown of this continuum hydrodynamics relation for molecular scale solutes has been noted in several previous experimental [38] , simulation [39] and theoretical [40] studies, and was also discussed as one possible explanation of the original experimental results on the viscosity dependence of helix-coil dynamics [13] . We have determined the diffusion coefficient of Lennard–Jones (LJ) particles in water from the mean-square displacement, using the parameters for an amide carbon atom in the Amber ff03 force field ( σ = σ 0 ≡0.373 nm), and an alternative model in which σ =2 σ 0 . In both cases, the diffusion coefficient, shown in Fig. 3a , shows a negligible deviation from the viscosity dependence expected from Stokes law, with the data for the larger particle being even closer to the expected D ∝ η −1 line. Note that this viscosity dependence does not confirm the validity of Stokes law for molecular solutes. However, even if molecules do not fulfil the requirements for the law to be valid, an inverse viscosity dependence of the diffusion coefficient is not unexpected, because the viscosity sets the time scale of solvent density fluctuations, which dominate condensed phase dynamics. 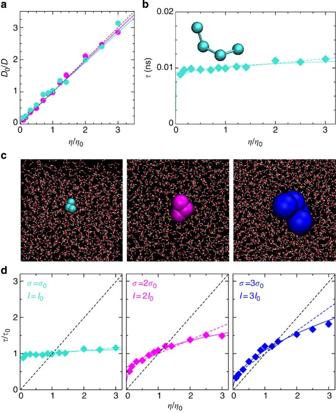Figure 3: Microscopic models. (a) Diffusion coefficient for single LJ particle in water. Cyan,σ=σ0; magenta,σ=2σ0, whereσ0is the LJσfor an sp2carbon in Amber ff03. (b) Viscosity-dependent isomerization rate for four-bead butane-like molecule forσ=σ0. (c) Illustrations of solute models used to study the effect of solute size on butane isomerization rate. (d) Scaling of transition times with solvent viscosity for the different set of parameters. Inaerrors were obtained by choosing alternative initial points for the fits of the mean squared displacement as a function of time. Elsewhere errors bars were obtained from bootstrap tests. Figure 3: Microscopic models. ( a ) Diffusion coefficient for single LJ particle in water. Cyan, σ = σ 0 ; magenta, σ =2 σ 0 , where σ 0 is the LJ σ for an sp 2 carbon in Amber ff03. ( b ) Viscosity-dependent isomerization rate for four-bead butane-like molecule for σ = σ 0 . ( c ) Illustrations of solute models used to study the effect of solute size on butane isomerization rate. ( d ) Scaling of transition times with solvent viscosity for the different set of parameters. In a errors were obtained by choosing alternative initial points for the fits of the mean squared displacement as a function of time. Elsewhere errors bars were obtained from bootstrap tests. Full size image Since single amino-acid residues are typically larger than 2 σ 0 , a deviation of diffusion coefficients from first-power dependence on viscosity is unlikely to be relevant here. An alternative possibility, suggested by the results for the alanine dipeptide, is that the friction is specifically associated with the isomerization of dihedral angles, rather than larger length-scale diffusive motion. This can be demonstrated more explicitly in a minimal model for dihedral transitions: a united-atom butane-like molecule, in which each of the atoms has the LJ parameters of an aliphatic carbon in the Amber ff03 force field (see Supplementary Methods and Supplementary Fig. 5 for details). Remarkably, we find that in this case, the transition rates between minima are almost independent of the solvent viscosity ( Fig. 3b ), an even stronger effect than observed for any of the peptides. This deviation persists even if the atoms of the butane molecule are increased to the size at which, in isolation, their diffusion coefficients would be almost perfectly proportional to inverse viscosity. ( Fig. 3c,d ), suggesting that torsional transition rates are intrinsically insensitive to the solvent friction. A role for torsional transitions in generating ‘internal friction’ in polymers was invoked in the earliest work on the subject [41] , although the molecular origin was not clear [42] . Solvent memory effects in the crossing of local barriers An explanation for the viscosity dependence of dihedral isomerization, predicted by Wolynes and co-workers [5] to be the cause of internal friction effects, involves the nature of the frictional forces exerted by the water molecules. In Kramers rate theory, the frictional forces are uncorrelated in time. For a molecular solvent, where the frictional forces are correlated, this can still be a good approximation if the correlation is lost quickly relative to the barrier crossing time. However, if the system crosses a local energy barrier on a comparable time scale to that of the solvent relaxation, a smaller frictional effect will in general be experienced. This could happen for very narrow or sharp energy barriers: torsional barriers, or other local barriers on the energy landscape, may fit this scenario. We investigate this effect quantitatively by considering a particle in a model energy landscape. We consider an LJ particle, solvated in explicit water, crossing the barriers of a one-dimensional (1D) external potential V ( x )= V 0 cos(2π nx / L x ) where x and L x are the Cartesian x coordinate of the particle and the box length in the x direction respectively, and we set V 0 =5 kJ mol −1 to obtain 10 kJ mol −1 barriers. Variation of the number of minima, n , systematically alters the barrier width and curvature. In Fig. 4a we show the dependence of the escape time on solvent viscosity for different n (the escape time is the mean time to escape from one minimum to one of its neighbours). It is clear that for increasing n (and hence barrier curvature), the mean barrier-crossing times become progressively less sensitive to solvent friction, suggesting that correlated friction, or memory friction, is significant. 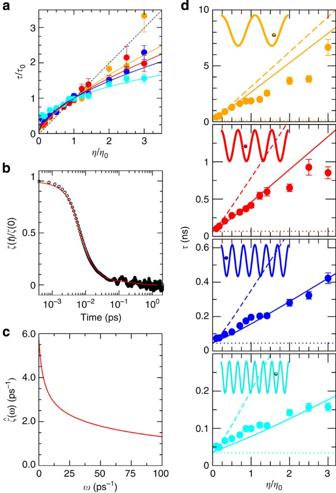Figure 4: Local barrier crossing rates for a particle in explicit water subject to a 1D external potential. (a) Viscosity dependence of (normalized) escape times for different numbers of miniman: orange, red, blue and cyan symbols correspond ton=2, 4, 6, 8, respectively. Curves are power-law fits. (b) Force autocorrelation functionζ(t) and (c) its Laplace transform. (d) Viscosity-dependent escape times for particle in potentials withn=2, 4, 6 and 8 (top to bottom) minima. Symbols are escape times from simulation, and solid, dashed and dotted lines represent respectively the predictions of Grote–Hynes, Kramers and transition-state theories. Insets illustrate the systems under consideration. Error bars were obtained from bootstrap tests. Figure 4: Local barrier crossing rates for a particle in explicit water subject to a 1D external potential. ( a ) Viscosity dependence of (normalized) escape times for different numbers of minima n : orange, red, blue and cyan symbols correspond to n =2, 4, 6, 8, respectively. Curves are power-law fits. ( b ) Force autocorrelation function ζ ( t ) and ( c ) its Laplace transform . ( d ) Viscosity-dependent escape times for particle in potentials with n =2, 4, 6 and 8 (top to bottom) minima. Symbols are escape times from simulation, and solid, dashed and dotted lines represent respectively the predictions of Grote–Hynes, Kramers and transition-state theories. Insets illustrate the systems under consideration. Error bars were obtained from bootstrap tests. Full size image The simplest model capturing the effect of memory friction is the Grote–Hynes rate theory for crossing a parabolic barrier [43] . In this theory, the rate is sensitive to the spectrum of relaxation times for forces operating on the reaction coordinate, determined by the Laplace transform of the autocorrelation function (or friction kernel) ζ ( t ) of solvent forces on the x coordinate. We obtained ζ ( t ) from simulations of a fixed particle [44] at the lowest solvent mass (for which statistical errors are smallest), and then ζ at other solvent masses by appropriately scaling time ( Supplementary Fig. 6 shows that independently determined ζ ( t ) are in good agreement with this scaling). The resulting correlation function ζ ( t ) and corresponding Laplace transform for the lowest solvent mass are shown in Fig. 4b,c . In Fig. 4d , we compare the observed escape times with those calculated from Grote–Hynes theory via the simulated correlation functions (details in Supplementary Text and Supplementary Table 2 ). In most cases, we obtain very good agreement, and importantly, the trend of increasing deviation from first-power viscosity dependence with increasing n . This agreement suggests that the effects of barrier anharmonicity [45] , captured in a more sophisticated rate theory [46] , are not needed in this case. For reference, we also show two other limits: (i) the transition-state theory rate, where solvent friction is ignored and (ii) the Kramers rate, in which friction is memoryless. The actual rate lies between these limits. For small n , the Kramers result is a good approximation, but becomes increasingly poor for large n . We note that an early molecular dynamics study of torsional isomerization also suggested that overdamped Kramers theory gave a poor description of the reaction dynamics, due to the slow time scale of solvent rearrangement [47] . We have chosen to study a simple model potential due to its generality, but its barriers can be approximately related to torsion barriers, by noting that the local curvature of the potential of mean force W ( ϕ ) for rotation about a torsion angle ϕ , projected onto direction of motion of the terminal atoms at the barrier top, x , is approximately , where r b is the radial separation of the terminal atoms from the axis of the central bond. This can be compared with the curvature in our 1D potential, (2π n / L x ) 2 V 0 . These calculations result in curvatures of 0.18, 0.41 and 1.62 J m −2 for the butane models with σ =3 σ 0 , 2 σ 0 , σ 0 respectively, and 0.13, 0.51, 1.15 and 2.05 J m −2 for the 1D models with n =2, 4, 6 and 8, respectively. Although a less direct comparison, the curvature of the alanine dipeptide barrier is ~1.72 J m −2 . The extent of deviation from the τ ∝ η line follows the variation in barrier curvature. Consistent with this, reducing the torsion barrier for Alanine dipeptide by 5 kJ mol −1 , reducing barrier curvature, results in a relaxation time whose dependence on viscosity is closer to first power ( Fig. 2c ). Crossing torsion barriers on folding transition paths There is a remarkably close correspondence between the overall relaxation times for short peptides and the local barrier crossing times in alanine dipeptide, which can be explained the memory friction effects discussed above. To extend these results to a larger system, we have studied the smallest protein for which internal friction has been experimentally characterized, Trp Cage tc5b (ref. 15 ). From multiple long simulations of this protein at 360 K, close to its folding midpoint temperature in simulation, we have determined an MSM as a function of solvent viscosity. Remarkably, we find a similar insensitivity to solvent viscosity to that observed for other systems ( Fig. 5a ). The exponents for a power-law fit to the dependence of relaxation times on viscosity are slightly smaller even than those at 300 K. A similar depenence of power-law exponent on temperature is observed for Ala dipeptide relaxation ( Supplementary Fig. 7 ), suggesting it may also originate at the level of individual torsion angles. 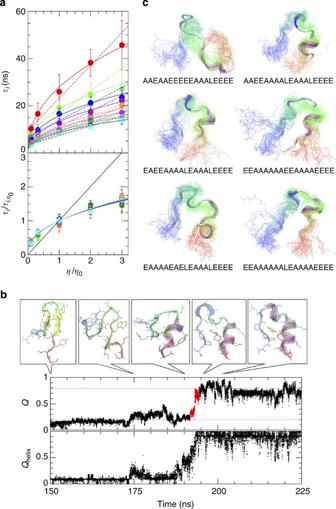Figure 5: All-atom folding dynamics of the Trp Cage tc5b. (a) Viscosity dependence of relaxation modes of Trp cage. Errors were obtained from bootstrap tests. (b) Example transition path showing formation of helical structureen routeto the native state. (c) Transition-state structures identified from a committor analysis of the Trp cage MSM. Figure 5: All-atom folding dynamics of the Trp Cage tc5b. ( a ) Viscosity dependence of relaxation modes of Trp cage. Errors were obtained from bootstrap tests. ( b ) Example transition path showing formation of helical structure en route to the native state. ( c ) Transition-state structures identified from a committor analysis of the Trp cage MSM. Full size image If torsional transitions, as in helix formation, are important in determining the dynamics near the folding transition state, we would expect to observe a variation in helix content on folding transition paths: specifically, helix formation should be important near the folding transition state. Of course, the helix has to be formed in order to fold, but alternative scenarios would be that it either is formed already at the start of the transition path, or (less likely) only forms at the very end. In Fig. 5b , we show a representative folding transition path for this protein. Notably, in the unfolded state, there is little helix content, and helix formation (tracked by the number of helical backbone contacts) is closely correlated with the overall folding (represented by the global fraction of native contacts); had the helix already been formed in the unfolded state, we would clearly be looking at a different scenario. By selecting states from our MSM with committors (or P fold values) in the range of 0.48–0.51 (details in Supplementary Methods ), we can zoom in on the folding transition states ( Fig. 5c ). These have in common the formation of a single alpha helical turn, clearly implying that the helix is in the process of being formed at the transition state. We have shown that the rates for crossing of local barriers can exhibit a strong deviation from inverse first-power dependence on solvent viscosity. This deviation can be attributed to the effects of solvent memory friction when the barrier crossing time is sufficiently fast. We note that earlier theoretical studies had also anticipated a power-law behaviour for crossing a barrier in the presence of memory friction [35] or fluctuating barriers [36] . How are these local barrier crossings related to global folding dynamics? For a small system like Ala 5 , where all of the relevant microscopic transitions can be approximated as single torsion transitions, this deviation approximately carries over to the global relaxation times via scaling of all microscopic rates. In temperature jump measurements on helical peptides [13] , a nearly single-exponential relaxation rate was observed, whose dependence on solvent viscosity is remarkably similar to what we find for Ala 5 (ref. 37 ; Fig. 6a ). Therefore, we can reasonably argue that this arises from a similar mechanism to that which we see for Ala 5 . Remarkably, after considering many possibilities, the authors of the experimental work came to the same conclusion [13] . While the comparison with experiment in the case of helical peptides is somewhat indirect, for the C(AGQ) 2 W peptide we can directly compute the relaxation rates measured experimentally for the same peptide, for which the finite rate of contact quenching needs to be considered [48] . The results of this calculation are overlaid with the experimental data in Fig. 6b , showing a good agreement. Contact formation rates in (Gly-Ser) n peptides reflect a similar internal friction effect [20] ( Supplementary Fig. 8 ). 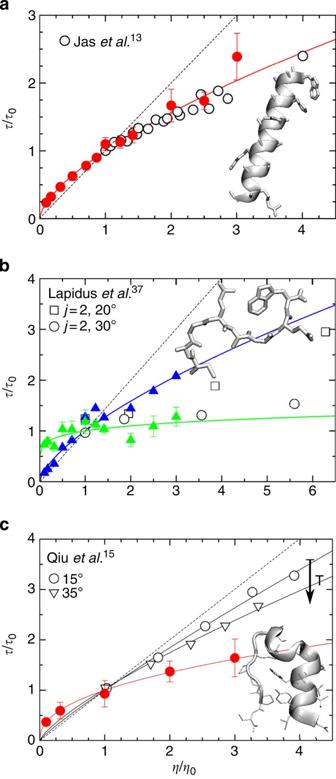Figure 6: Comparison with experimental viscosity dependence. (a) Normalized relaxation times from temperature-jumps to 293 K on the WAAAH+-(AAARA)3A peptide, digitized fromref.13and results from simulation of Ala5(red circles). (b) Comparison of quenching rates from the diffusion-limited scenario and the full calculation with the experimental data for the C(AGQ)2W peptide37. (c) Comparison of slowest mode of trpcage (red) with folding rates at different temperatures15, marked with different symbols. Black lines mark the power law fits to the experimental data, with gradually decreasing exponents.. Figure 6: Comparison with experimental viscosity dependence. ( a ) Normalized relaxation times from temperature-jumps to 293 K on the WAAAH + -(AAARA) 3 A peptide, digitized fromref. [13] and results from simulation of Ala 5 (red circles). ( b ) Comparison of quenching rates from the diffusion-limited scenario and the full calculation with the experimental data for the C(AGQ) 2 W peptide [37] . ( c ) Comparison of slowest mode of trpcage (red) with folding rates at different temperatures [15] , marked with different symbols. Black lines mark the power law fits to the experimental data, with gradually decreasing exponents.. Full size image How far can our results be extended to larger proteins? The case of Trp Cage, discussed above, provides a minimal example. Both the experimental and simulated viscosity-dependent relaxation times deviate from first-power viscosity dependence ( Fig. 6c ). The power-law exponent is smaller in the simulations, but this is most likely related to the higher temperature (360 K)—a change in exponent was already evident when the experimental temperature was varied from 288 to 308 K ( Fig. 6c ). A similar change in the villin headpiece subdomain has been attributed to a shift in the transition state with temperature [16] . An additional contribution may come from dihedral barrier crossings, as increasing temperature also reduces the viscosity dependence of alanine dipeptide isomerization. For larger chains, one can no longer simply assume a global scaling of all microscopic rates, because hydrodynamic effects will start to become important for some transitions. In fact, even for the Ala 5 peptide, the slower modes are systematically more sensitive to viscosity than the fast ones, presumably because they involve more global rearrangements ( Fig. 1f )—as predicted theoretically [5] . For larger proteins, an alternative perspective would consider folding as diffusion along a global folding coordinate, for example, the fraction of native contacts, Q (refs 6 , 49 , 50 ). If crossing of local barriers is the dominant contribution to the diffusion coefficient along the global coordinate at the folding transition state (as for Trp Cage), then it would be expected that the viscosity dependence of the global diffusion coefficient (and hence folding rate) would scale with solvent viscosity in a similar way to the local barriers [6] . This is analogous to the variation of diffusion coefficients with viscosity in a jump-diffusion model [51] , in which the dynamics along the global coordinate arises from hopping between many local minima, and the diffusion coefficient is proportional to the hopping rate. This reasoning also justifies the use of Kramers theory to describe the global folding reaction, even when it may not adequately describe local transitions on the landscape. On the other hand, if large-scale motion of the chain through the solvent is more important than dihedral isomerization near the transition state, one would expect the diffusion coefficient on the folding coordinate to more closely follow an inverse first-power viscosity dependence. In addition to Trp Cage, we do indeed find that many other proteins follow a similar trend to the peptide models. Examples include the helical protein cytochrome c 14 , or villin HP35 at low temperatures [16] ( Supplementary Fig. 9 ). In these cases, we suggest that the folding dynamics is dominated by helix formation and so the viscosity dependence of the folding diffusion coefficient is determined by that of the individual torsion transitions. However, there are other examples in which internal friction is less evident than for helix formation, for example the folding of cold-shock protein, the GB1 hairpin or spectrin R15, or the reconfiguration dynamics of proteins in high denaturant concentration follow a near first-power dependence on viscosity. This is reminiscent of the more ideal behaviour we find for the coarse-grained helical protein, relative to dihedral transitions in the same model. That could be rationalized if, for example, the diffusion coefficient at the top of the folding barrier is more sensitive to the mutual diffusion of secondary structure elements than on torsional transitions. This may be one reason why experimental evidence for internal friction effects is more frequently found for small or helix-rich proteins [13] , [14] , [15] , [16] , [18] than for large or non-helical ones in which chain diffusion may be more important [8] , [9] , [27] , [52] . On the other hand, several examples, such as unfolded proteins [19] in low denaturant, or the folding of α 3 D (ref. 34 ) or the spectrin R16 and R17 domains [10] , exhibit stronger evidence of internal friction (as assessed by deviation from the line τ ∝ η ) than our peptide models (see, for example, the spectrin data in Supplementary Fig. 9 ). It seems unlikely in these cases that torsional transitions can be the only explanation for the unusual viscosity dependence, as amino acid dipeptides with both small (glycine dipeptide) and large (tryptophan dipeptide) side-chains have relaxation rates with viscosity dependence very similar to that for alanine dipeptide ( Supplementary Fig. 10 ). Since dipeptides can be considered as minimal models for torsion angle transitions, torsional barriers are unlikely to be the only source of the internal friction observed for these proteins. Other sources may include memory friction for a different kind of local energy barrier, for example, reptation between different helix registers [34] , [53] ; or an alternative internal friction mechanism, perhaps due to shielding of the chain from the solvent. For example, greater friction emerges for more compact unfolded states at low denaturant [17] , [19] , and for the Villin headpiece subdomain at higher temperature, where the folding transition state becomes more native-like. By changing viscosity using the solvent mass in our simulations, we simplify the interpretation, but we consequently do not include some factors which have been implicated in the experimental interpretation. For example, one suggested origin of (apparent) internal friction effects in protein-folding experiments is a difference in protein:solvent interactions as a function of solution composition, leading to a change of free energy surface [54] . Our results show that internal friction effects can arise even when the free energy surface is identical, since our energy function is not altered, although this of course does not rule out that changes in free energy surface are relevant experimentally. An additional factor to bear in mind is the nature of the experimental solvent, which is usually a solution of a viscogen (and possibly chaotropes such as urea or guanidinium chloride) of similar size to amino-acid residues. It might seem that describing the solvent friction on a peptide arising from such complex solutions by a single viscosity parameter is an oversimplification, and possible differences between the macroscopic solution viscosity (‘macroviscosity’) and the effective viscosity (‘microviscosity’) experienced by the protein have been discussed [11] , [55] . However, we find that the viscosity-dependent torsion isomerization rates obtained by varying glucose concentration are almost identical to those measured by varying solvent mass. Therefore, the torsion angle friction identified in this work should also be relevant to experiments using chemical viscogens. In conclusion, we have used a series of molecular models of varying complexity to investigate possible origins of internal friction evident in an idealized situation in which only the solvent viscosity, and not protein–solvent interactions, are varied. Any deviation of translational diffusion coefficients from a Stokes-like dependence on solvent viscosity for very small solutes is too small an effect to explain the observed internal friction effects on relaxation rates. Instead, we find that the insensitivity of peptide dynamics and folding to solvent viscosity can be ascribed to the local ‘roughness’ of the energy landscape, involving the crossing of torsion angle barriers, such that memory friction effects become important. This suggests that variation of solvent viscosity is complementary to variation of temperature or mechanical force as a means of probing landscape roughness [56] , [57] . The mechanism we find can directly explain the internal friction effects observed in helical peptides and the helical Trp Cage miniprotein, and most likely explains, via its effect on the folding diffusion coefficient, internal friction in some larger helical proteins. Possible additional sources of internal friction in other situations remain to be elucidated. Atomistic MD simulations MD simulations were run using the Amber ff03 (ref. 58 ) or ff03* (ref. 59 ) force fields in explicit water, in the isothermal–isobaric ensemble. Viscosity was varied by altering the solvent mass, and the integration time step adjusted accordingly. Markov state models Simulation data were analysed using an MSM [60] , with discrete states being based on the values of the five backbone torsion angles, with α and β/PPII regions being defined as shown in Fig. 1b . This results in two possibilities for each amino acid and a total of 2 5 =32 for the whole Ala 5 peptide [32] , [33] . For Trp Cage, additional states were added to describe the conformations of the glycine residues ( Supplementary Fig. 11 and Supplementary Table 3 ). For simplicity, in this case we calculate the transition probability matrix T (Δ t ) using the maximum-likelihood estimator T ji = N ji /Σ j N ji (ref. 61 ), where N ji is the number of transitions from micro-state i to micro-state j observed in the simulation trajectory for an observation (lag) time Δ t . The transition matrix has 32 eigenvalues, λ i , and from them we can obtain the characteristic relaxation times as τ i =−Δ t /ln( λ i ). Each of these corresponds to a exchange of population between the states in the discretized space. Full details of simulations and other methods are given in Supplementary Information. How to cite this article: de Sancho, D. et al . Molecular origins of internal friction effects on protein-folding rates. Nat. Commun. 5:4307 doi: 10.1038/ncomms5307 (2014).